Val66Met polymorphism of BDNF alters prodomain structure to induce neuronal growth cone retraction A common single-nucleotide polymorphism (SNP) in the human brain-derived neurotrophic factor ( BDNF ) gene results in a Val66Met substitution in the BDNF prodomain region. This SNP is associated with alterations in memory and with enhanced risk to develop depression and anxiety disorders in humans. Here we show that the isolated BDNF prodomain is detected in the hippocampus and that it can be secreted from neurons in an activity-dependent manner. Using nuclear magnetic resonance spectroscopy and circular dichroism, we find that the prodomain is intrinsically disordered, and the Val66Met substitution induces structural changes. Surprisingly, application of Met66 (but not Val66) BDNF prodomain induces acute growth cone retraction and a decrease in Rac activity in hippocampal neurons. Expression of p75 NTR and differential engagement of the Met66 prodomain to the SorCS2 receptor are required for this effect. These results identify the Met66 prodomain as a new active ligand, which modulates neuronal morphology. A common single-nucleotide polymorphism (SNP) in the human brain-derived neurotrophic factor ( BDNF ) gene is highly associated with abnormalities in episodic memory, a reduction in the hippocampal volume and enhanced risk for depression and anxiety disorders in humans [1] , [2] , [3] , [4] , [5] , [6] , [7] , [8] . This SNP (rs6265) is observed in more than 25% of the human population (Database of Single-Nucleotide Polymorphisms-National Center for Biotechnology Information, National Library of Medicine, 2012), and it leads to a nucleotide change from a guanine to an adenine at position 196 (G196A) that results in a valine (Val) to methionine (Met) substitution at codon 66 (Val66Met). BDNF is translated as a precursor protein (proBDNF) consisting of an amino-terminal prodomain and a carboxy-terminal mature domain (mBDNF). The Val66Met substitution site is within the prodomain ( Supplementary Fig. S1 ). ProBDNF can be cleaved by furin or proconvertases in the trans-Golgi network or secretory vesicles, respectively [9] . Both mBDNF and proBDNF can be secreted from neurons [10] , [11] in an activity-dependent manner after KCl-induced depolarization [10] or electrical stimulation [11] . In addition, proBDNF can be cleaved extracellularly by plasmin generated by tissue plasminogen activator or by selective matrix metalloproteinases including MMP3, MMP7 (ref. 12 ) and MMP9 (ref. 13 ) to release mBDNF. The fate of the isolated BDNF prodomain after proBDNF intracellular or extracellular proteolysis is not known. mBDNF binds the tropomyosin-related kinase B receptor to promote neuronal survival, differentiation, neurogenesis and synaptic plasticity. Modest changes in mBDNF levels in rodents result in alterations in the hippocampal function and behavioural abnormalities. In contrast, uncleaved proBDNF promotes apoptosis by binding to a receptor complex of p75 neurotrophin receptor (p75 NTR ) and sortilin (a Vps10p-domain sorting receptor family member) [14] . Interestingly, recent reports have shown that proBDNF [15] as well as unprocessed pro-nerve growth factor (proNGF) [16] induce growth cone retraction in cultured neurons. The BDNF prodomain is highly conserved with a valine at or near position 66 in more than 70 species examined to date ( Supplementary Fig. S1 ). The prodomain mediates an interaction with sortilin [17] , which acts as a chaperone to direct intracellular trafficking of proBDNF to the regulated secretory pathway. The Met66 proBDNF variant exhibits decreased binding to sortilin, altered intracellular trafficking and a reduction in the activity-dependent secretion of mBDNF [2] , [6] , [17] , [18] . Moreover, a knock-in mouse that expresses Met66 BDNF recapitulates many specific phenotypic properties of the human polymorphism [6] . Thus, the proposed mechanism by which Met66 BDNF mediates central nervous system effects is indirect, by a reduction in activity-dependent release of mBDNF leading to altered synaptic plasticity. However, the high-sequence conservation of the BDNF prodomain ( Supplementary Fig. S1 ), and the recent evolutionarily emergence of the Val66Met polymorphism (only present in humans) prompted us to ask whether the isolated prodomain might function as an independent ligand. We have found that the prodomain is present at high levels in vivo and is secreted from neurons in an activity-dependent manner. We further considered whether the Val66 and Met66 prodomains exhibit different structures to elicit distinct biological activities. Here we show that structural changes induced by Val66Met substitution confer bioactivity to the prodomain, as only the Met66 prodomain acutely alters neuronal morphology. Finally, we demonstrate that the prodomain exerts this effect through differential interaction with SorCS2, the sortilin-related Vps10p-domain sorting receptor 2. Our findings suggest that the Met66 prodomain activity is an additional mechanism that may contribute to the increased incidence of depression and anxiety disorders found in humans with the SNP. BDNF prodomain is expressed in the hippocampus and secreted The hippocampus is a key regulator of learning and memory and dysfunction of its neural circuitry underlies the development of memory impairment, depression and anxiety disorders [19] . To determine if the BDNF prodomain may affect the structure of hippocampal neurons, we first examined whether the prodomain was present in this brain region. Detection of the isolated prodomain in vitro and in vivo has been technically challenging due to low antibody sensitivity. However, glutaraldehyde fixation of proteins to the transfer membranes following sodium dodecyl sulphate polyacrylamide gel electrophoresis (SDS–PAGE), and the use of a BDNF prodomain-specific monoclonal antibody previously characterized [10] , facilitated its detection in the mouse hippocampus as a 15.5 kDa band ( Fig. 1a ). In order to demonstrate specificity of detection, we observed that the prodomain levels are reduced by half in Bdnf heterozygous ( Bdnf +/− ) mouse hippocampal lysates compared with wild-type (WT) littermates ( Fig. 1b ). As the prodomain contains an N -linked glycosylation site ( Supplementary Fig. S1 ), we performed enzymatic removal of the N -linked glycosylation, which resulted in migration of the prodomain at 12.3 kDa, consistent with the predicted molecular weight by its amino-acid sequence ( Fig. 1c ). 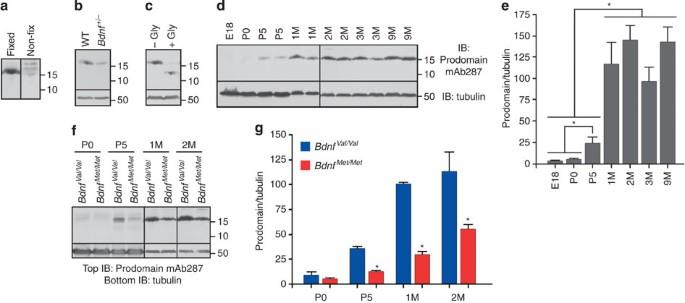Figure 1:The BDNF prodomain is detected at high levelsin vivo. (a) Detection of BDNF prodomain (15.5 kDa.) from mice hippocampus after glutaraldehyde fixation of the transfer membrane following SDS–PAGE. (b) The prodomain levels were reduced by half inBdnf+/−mice hippocampal lysates, compared with WT. (c) Treatment of the hippocampal lysates withN-glycanase (+Gly) reduced the molecular weight of the prodomain to 12.3 kDa. (d) BDNF prodomain levels at embryonic day 18 (E18), postnatal days 0 and 5 (P0 and P5), and 1, 2, 3 or 9 months (M) in hippocampal lysates of C57BL/6 mice. (e) Quantification of (d). Bars represent mean±s.e.m. of prodomain densitometry data normalized to β tubulin;n=3 per group. (f) Comparison of BDNF prodomain levels from hippocampi ofBdnfVal/ValandBdnfMet/Metmice at P0, P5, 1 and 2 months of age. (g) Quantification of (f). Bars represent mean±s.e.m. of prodomain densitometry data normalized to β tubulin;n=4 per group. Statistical comparisons were made by one-way analysis of variance test. *P<0.05. Figure 1: The BDNF prodomain is detected at high levels in vivo . ( a ) Detection of BDNF prodomain (15.5 kDa.) from mice hippocampus after glutaraldehyde fixation of the transfer membrane following SDS–PAGE. ( b ) The prodomain levels were reduced by half in Bdnf +/− mice hippocampal lysates, compared with WT. ( c ) Treatment of the hippocampal lysates with N -glycanase (+Gly) reduced the molecular weight of the prodomain to 12.3 kDa. ( d ) BDNF prodomain levels at embryonic day 18 (E18), postnatal days 0 and 5 (P0 and P5), and 1, 2, 3 or 9 months (M) in hippocampal lysates of C57BL/6 mice. ( e ) Quantification of ( d ). Bars represent mean±s.e.m. of prodomain densitometry data normalized to β tubulin; n =3 per group. ( f ) Comparison of BDNF prodomain levels from hippocampi of Bdnf Val/Val and Bdnf Met/Met mice at P0, P5, 1 and 2 months of age. ( g ) Quantification of ( f ). Bars represent mean±s.e.m. of prodomain densitometry data normalized to β tubulin; n =4 per group. Statistical comparisons were made by one-way analysis of variance test. * P <0.05. Full size image During late embryonic and early postnatal murine development, the expression of the prodomain in the hippocampus of C57BL/6 mice was negligible ( Fig. 1d,e ). However, the prodomain was detected at postnatal day 5, its expression increased significantly at 1 month and plateaued in adult mice (3–9 months) ( Fig. 1d,e ). The prodomain was detectable in the hippocampi of both WT Bdnf Val/Val and Bdnf Met/Met knock-in animals [6] . However, the levels of expression significantly differ, as Bdnf Met/Met mice displayed lower levels of expression as compared with Bdnf Val/Val in all the time points studied ( Fig. 1f,g ). Other commercially available antibodies to the prodomain of BDNF (ANT-006, Alomone, Jerusalem, Israel) failed to detect the endogenous prodomain in isolation and showed very low sensitivity in detecting the recombinant prodomains ( Supplementary Fig. S2 ). To determine if the prodomain was secreted, we cultured the rat hippocampal neurons in conditions to reduce glia contamination and collected the conditioned media of day 6 in vitro (DIV6) cultures. The endogenous prodomain was detected in the media, and prodomain levels were increased significantly after depolarization with 25 mM KCl for 6 h ( Fig. 2a,b ). Lactate dehydrogenase (LDH) assays demonstrated there was no significant release by the cells under these culture conditions after depolarization with KCl (arbitrary LDH release units: control 0.21±0.01; KCl 0.20±0.01). Incubation of the hippocampal neuron cultures from DIV3 to DIV6 with α-2-anti-plasmin and/or MMP inhibitor II (which inhibits MMP1, 3, 7 and 9) to prevent extracellular cleavage of secreted proBDNF did not significantly alter the levels of the prodomain secreted in the media in basal conditions or after depolarization ( Fig. 2a,b ). Enzymatic removal of N -linked glycosylation resulted in a reduction of the molecular mass of the endogenous secreted prodomain from 15.5 kDa to the predicted 12.3 kDa ( Fig. 2c ) as described above for the prodomain expressed in the hippocampus. We next compared the activity-dependent secretion of the prodomain from hippocampal–cortical cultures obtained from Bdnf Val/Val and Bdnf Met/Met knock-in mice [6] . We found that both Val66 and Met66 prodomains can be secreted after depolarization with KCl; however, the levels of secreted Met66 prodomain were significantly lower as compared with the Val66 prodomain ( Fig. 2d,e ). These results suggest that the prodomain is detectable in the adolescent and adult murine hippocampus and that neurons secrete it. 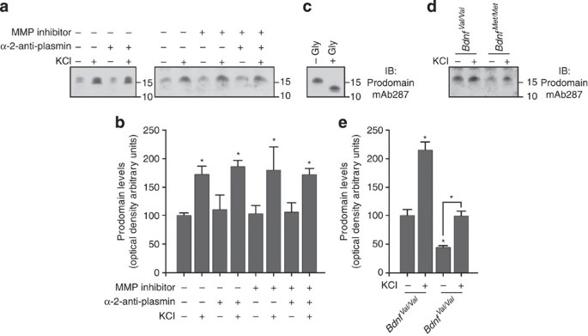Figure 2: The BDNF prodomain is secreted from cultured neurons. (a) Prodomain was detected in the media of DIV6 rat hippocampal cultures. Cultures were treated with or without α-2 anti-plasmin and/or MMP inhibitor II (MMP1, 3, 7 and 9 inhibitor) in order to prevent extracellular cleavage of secreted proBDNF. Activity-dependent secretion was achieved by depolarization with KCl. (b) Quantification of (a). Bars represent mean±s.e.m. of prodomain densitometry data;n=3 per group. (c) Treatment withN-glycanase reduced the molecular mass of the secreted prodomain. (d) Prodomain was detected in the media of DIV6 hippocampal–cortical neurons from E18 pups obtained fromBdnfMet/+xBdnfMet/+mice litters. Level of secreted prodomain differ betweenBdnfVal/ValandBdnfMet/Metcultures. (e) Quantification of (d). Bars represent mean±s.e.m. of prodomain densitometry data;n=4 per group. Statistical comparisons were made by one-way analysis of variance test. *P<0.05. Figure 2: The BDNF prodomain is secreted from cultured neurons. ( a ) Prodomain was detected in the media of DIV6 rat hippocampal cultures. Cultures were treated with or without α-2 anti-plasmin and/or MMP inhibitor II (MMP1, 3, 7 and 9 inhibitor) in order to prevent extracellular cleavage of secreted proBDNF. Activity-dependent secretion was achieved by depolarization with KCl. ( b ) Quantification of ( a ). Bars represent mean±s.e.m. of prodomain densitometry data; n =3 per group. ( c ) Treatment with N -glycanase reduced the molecular mass of the secreted prodomain. ( d ) Prodomain was detected in the media of DIV6 hippocampal–cortical neurons from E18 pups obtained from Bdnf Met/+ x Bdnf Met/+ mice litters. Level of secreted prodomain differ between Bdnf Val/Val and Bdnf Met/Met cultures. ( e ) Quantification of ( d ). Bars represent mean±s.e.m. of prodomain densitometry data; n =4 per group. Statistical comparisons were made by one-way analysis of variance test. * P <0.05. Full size image Val66Met substitution alters the BDNF prodomain structure To evaluate if there are structural differences in the Val66 and Met66 prodomains, we produced both human recombinant prodomains in Escherichia coli (residues 23–113 displayed in red in Supplementary Fig. S1 ). The purity of the recombinant prodomains was examined by Coomassie blue and silver staining ( Supplementary Fig. S3a,b ). By SDS–PAGE, the recombinant prodomains migrate at the predicted molecular weight of 10.2 kDa, with no difference in the detection of the Val66 and Met66 prodomains by the specific prodomain antibody used ( Supplementary Fig. S3c ). The BDNF prodomain is predicted to be disordered by structure prediction software ( Supplementary Fig. S4 ). This predicted disorder in the BDNF prodomain is consistent with the absence of a defined trace of the related nerve growth factor prodomain in the proNGF-p75 NTR crystal lattice, indicating a lack of ordered structure [20] . To define the structural effects of the Val66Met polymorphism, we examined the Met66 and Val66 prodomains using nuclear magnetic resonance (NMR). The 1 H– 15 N heteronuclear correlation spectra indicated that the Val66 and Met66 prodomains are intrinsically disordered, lacking stable secondary or tertiary structure ( Fig. 3 , Supplementary Fig. S5 ). Secondary chemical shifts analysis for the Val66 prodomain and the Met66 prodomain indicate that both are primarily disordered structures ( Supplementary Fig. S6 ). Moreover, in the NMR conditions employed, both prodomains were monomeric showing no evidence of oligomerization or concentration-dependent change in spectral properties (from 2 to 450 μM). To define precise Val66Met structural differences, we generated sequence specific 1 H/ 13 C/ 15 N heteronuclear NMR assignments for the Val66 and Met66 prodomains using established triple-resonance NMR methods [21] . This technique assigns individual resonance frequencies to specific atoms within each amino acid in the prodomain sequence (chemical shifts displayed as peaks in Fig. 3a and Supplementary Fig. S5a,b ). The NMR chemical shifts provide a sensitive indicator of conformational preference within disordered states. Comparison of chemical shift deviations between the Val66 prodomain and the Met66 prodomain indicated that there are significant changes localized to seven residues (E64, H65, I67, E68, E69, L70, L71) neighbouring the Val66Met substitution site ( Fig. 3a,b ). The backbone chemical shifts for the prodomains are deposited in the Biological Magnetic Resonance Bank: Val66 ID number: 19358; Met66 ID number: 19357. 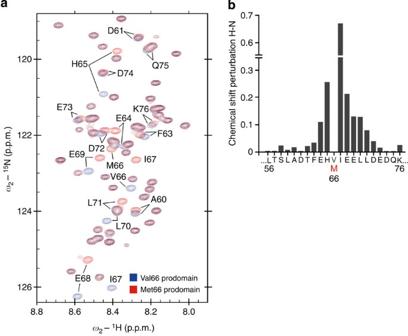Figure 3: Impact of the Val66Met substitution on the structure of the BDNF prodomain. (a) Overlay of the heteronuclear single-quantum coherence (HSQC) spectrum on the Val66 (blue) and Met66 (red) prodomains. Each cross-peak (chemical shift) corresponds to one residue within the sequence of the prodomain (one chemical shift for each covalently bonded pair of1H–15N atoms assigned to specific amides within the prodomain sequence). Full HSQC spectra of Val66 and Met66 prodomains are available inSupplementary Fig. S5. The backbone chemical shifts for the prodomains are deposited in the Biological Magnetic Resonance Bank: Val66 ID number: 19358. Met66 ID number: 19357. (b) Chemical shift deviation (Δδ) between BDNF Val66 and Met66 prodomains showed that changes induced by the substitution are localized to seven residues (E64, H65, I67, E68, E69, L70, L71) neighbouring the Val66Met substitution site. The variation in Δδ for residues 23–55, and 77–113 outside the display window was between 0.007 and 0.0037, p.p.m. Figure 3: Impact of the Val66Met substitution on the structure of the BDNF prodomain. ( a ) Overlay of the heteronuclear single-quantum coherence (HSQC) spectrum on the Val66 (blue) and Met66 (red) prodomains. Each cross-peak (chemical shift) corresponds to one residue within the sequence of the prodomain (one chemical shift for each covalently bonded pair of 1 H– 15 N atoms assigned to specific amides within the prodomain sequence). Full HSQC spectra of Val66 and Met66 prodomains are available in Supplementary Fig. S5 . The backbone chemical shifts for the prodomains are deposited in the Biological Magnetic Resonance Bank: Val66 ID number: 19358. Met66 ID number: 19357. ( b ) Chemical shift deviation (Δδ) between BDNF Val66 and Met66 prodomains showed that changes induced by the substitution are localized to seven residues (E64, H65, I67, E68, E69, L70, L71) neighbouring the Val66Met substitution site. The variation in Δδ for residues 23–55, and 77–113 outside the display window was between 0.007 and 0.0037, p.p.m. Full size image Val66 and Met66 prodomains transient secondary structure We estimated the prodomain secondary structure tendency based on the heteronuclear chemical shifts using the secondary structure propensity (SSP) score [22] . The positive SSP scores estimate regions of helical preference, whereas the negative scores indicate the residues with β-structure propensity. Upon Val66Met substitution, a shift in conformation from β-strand to helical conformation was observed around the position 66 ( Fig. 4a ). Outside the substitution area, the Val66 and Met66 prodomain SSP scores were coincident with regions of transient helix centred at residues 24, 44, 57 and 90, and β-structure that appears neighbouring residues 32, 50, 80, 101 and 110 ( Fig. 4a ). Chemical shift analysis using Talos+ secondary structure analysis software [23] showed a strong preference for β-strand around position 66 in the Val66 prodomain. The Met66 prodomain has reduced tendency to adopt β-strand as compared with the Val66 prodomain ( Fig. 4b,c ) consistent with the SSP score analysis. 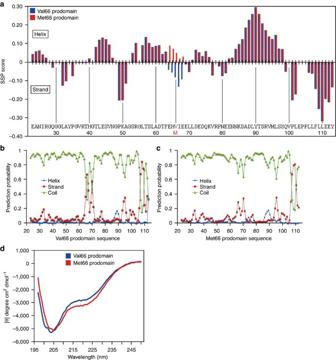Figure 4: Val66 and Met66 prodomains differ in transient secondary structure. (a) SSP score obtained using the backbone1H,15N,13C chemical shifts from the BDNF prodomain Val66 (blue bars) and Met66 (red bars). The SSP score identified regions of transient structure formation (positive values=α-helix, negative values=β-sheet). (b,c) Graphs illustrating secondary structure prediction by TALOS+ analysis using the heteronuclear backbone chemical shifts of Val66 (b) and Met66 (c) prodomains. α-helix in blue spheres, β-strand in red squares and disorder in green triangles. TALOS+ analysis showed decreased β-sheet propensity in the Met66 prodomain compared with the Val66 prodomain, result that is consistent with the SSP score. (d) Ultraviolet circular dichroism (CD) spectra of 30 μM of the Val66 (blue) and Met66 (red) prodomains collected in 10 mM NaH2PO4and 50 mM NaCl pH 7.0 at 23 °C. The negative peak around 200 nm revealed the natively unfolded conformation of both prodomains. However, the lower absorption at 222 nm for Met66 prodomain is consistent with increased tendency to helical conformation compared with the Val66 prodomain. Each spectrum is representative of four averaged scans and is normalized to the spectrum of buffer alone. Figure 4: Val66 and Met66 prodomains differ in transient secondary structure. ( a ) SSP score obtained using the backbone 1 H, 15 N, 13 C chemical shifts from the BDNF prodomain Val66 (blue bars) and Met66 (red bars). The SSP score identified regions of transient structure formation (positive values=α-helix, negative values=β-sheet). ( b , c ) Graphs illustrating secondary structure prediction by TALOS+ analysis using the heteronuclear backbone chemical shifts of Val66 ( b ) and Met66 ( c ) prodomains. α-helix in blue spheres, β-strand in red squares and disorder in green triangles. TALOS+ analysis showed decreased β-sheet propensity in the Met66 prodomain compared with the Val66 prodomain, result that is consistent with the SSP score. ( d ) Ultraviolet circular dichroism (CD) spectra of 30 μM of the Val66 (blue) and Met66 (red) prodomains collected in 10 mM NaH 2 PO 4 and 50 mM NaCl pH 7.0 at 23 °C. The negative peak around 200 nm revealed the natively unfolded conformation of both prodomains. However, the lower absorption at 222 nm for Met66 prodomain is consistent with increased tendency to helical conformation compared with the Val66 prodomain. Each spectrum is representative of four averaged scans and is normalized to the spectrum of buffer alone. Full size image In order to corroborate the SSP analysis and Talos+ results with an NMR-independent technique, we performed circular dichroism (CD) spectroscopy. The negative peak around 200 nm for both prodomains CD spectra revealed the predominant natively unfolded conformation, whereas the changes in CD intensity at 222 nm are characteristic of helix propensity ( Fig. 4d ). Met66 prodomain CD spectra showed a more negative absorption at 222 nm consistent with an increased helical tendency as compared with the Val66 prodomain ( Fig. 4d ), a result that is in agreement with the SSP and Talos+ data. To summarize, both NMR and CD analysis demonstrate that the Val66 prodomain has increased tendency to β-structure in the residues adjacent to the position 66, whereas the Met66 prodomain displays increased helical propensity. BDNF Met66 prodomain induces growth cone retraction The formation of neuronal networks depends upon the growth and retraction of nascent neuronal processes. Alterations in synaptic network organization influence the occurrence and progression of neuropsychiatric disorders [19] , [24] . Therefore, we assessed the bioactivity of Val66 and Met66 prodomains in mediating acute morphological changes in the hippocampal neurons using a growth cone retraction assay [16] . Unprocessed proNGF has been recently identified as a ligand that initiates acute retraction of growth cones, an effect mediated by the expression of p75 NTR and SorCS2, a member of the sortilin family of receptors [16] . A recent study indicates that proBDNF also induces growth cone retraction [15] , an effect that we have confirmed ( Supplementary Fig. S7a ). Thus, we examined whether BDNF prodomain in isolation could induce the same effect. We treated primary mouse hippocampal neurons with recombinant Val66 or Met66 prodomains. Surprisingly, the Met66 prodomain-induced rapid growth cone retraction over a period of 20 min, while the Val66 prodomain was inactive ( Fig. 5a,b ). This effect was achieved with 1 nM (10 ng ml −1 ) concentration of the Met66 prodomain. At 50 ng ml −1 , the Val66 prodomain also remained inactive without showing significant growth cone retraction ( Supplementary Fig. S8 ). As with proNGF [16] and proBDNF [15] ( Supplementary Fig. S7a ), the growth cone retraction effect induced by the Met66 prodomain was limited to p75 NTR -positive cells within the culture ( Fig. 5b ). 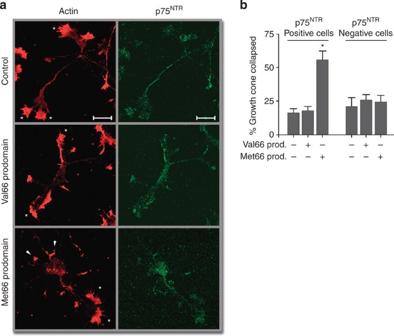Figure 5: The Met66 prodomain induces growth cone retraction in cultured hippocampal neurons. (a) Neurons were treated with Val66 or Met66 prodomains (10 ng ml−1) for 20 min, fixed and stained for actin and p75NTR. Arrows indicate retracted growth cones; asterisks indicate intact growth cones. Scale bar, 20 μm. (b) Quantification of growth cone retraction in p75NTR-positive cells shown in (a), compared with p75NTR-negative cells. Prodomain abbreviated as prod. (b)n=4 independent experiments. Bars represent mean±s.e.m. Statistical comparisons were made by one-way analysis of variance test. *P<0.05. Figure 5: The Met66 prodomain induces growth cone retraction in cultured hippocampal neurons. ( a ) Neurons were treated with Val66 or Met66 prodomains (10 ng ml −1 ) for 20 min, fixed and stained for actin and p75 NTR . Arrows indicate retracted growth cones; asterisks indicate intact growth cones. Scale bar, 20 μm. ( b ) Quantification of growth cone retraction in p75 NTR -positive cells shown in ( a ), compared with p75 NTR -negative cells. Prodomain abbreviated as prod. ( b ) n =4 independent experiments. Bars represent mean±s.e.m. Statistical comparisons were made by one-way analysis of variance test. * P <0.05. Full size image Met66 prodomain binds differentially to SorCS2 Prior experiments have established that p75 NTR and sortilin interact to form a receptor complex on the cell surface [25] , and that SorCS2 facilitates the interaction of p75 NTR with downstream signalling proteins to promote growth cone retraction [16] . We were unable to detect sortilin in these culture conditions, but SorCS2 was expressed in p75 NTR -positive cells [16] . Thus, we tested whether the prodomain interacts with SorCS2 and p75 NTR using co-immunoprecipitation analysis of cells expressing the prodomain with either of the receptors. We were unable to detect interaction of the prodomains with p75 NTR ( Fig. 6a ). However, both Met66 and Val66 prodomains interact with SorCS2 ( Fig. 6b ). By quantitative analysis, the Met66 prodomain interacted more effectively with SorCS2 than the Val66 prodomain ( Fig. 6b,c ). Moreover, we performed NMR spectroscopy of the Val66 prodomain or the Met66 prodomains with human recombinant SorCS2 to determine if the prodomains interacted differently with this receptor. Consistent with the co-immunoprecipitation result, both Val66 and Met66 prodomains interacted with SorCS2 as detected by chemical shift perturbation in the prodomains upon addition of the receptor ( Fig. 6d , Supplementary Fig. S9a,b ). Amino acids 34, 38–40, 51, 53–54, 76–77, 80, 96 and 100–111 of both Val66 and Met66 prodomains interact with SorCS2 as shown by chemical shift deviation upon addition of the receptor ( Fig. 6d ). Surprisingly, the Met66 prodomain displayed greater chemical shift changes upon interaction to SorCS2 between residues 65 and 71, whereas the same residues in the Val66 prodomain do not engage the receptor ( Fig. 6d , under #). This represents a novel region of interaction in the prodomain that is conferred by the Met66 substitution. These larger chemical shift changes in the Met66 prodomain upon SorCS2 binding may reflect a tighter interaction or a different binding conformation. Thus, although both prodomains interact with SorCS2, the interactions are distinct, and this difference can result in the differential activity of the prodomains. 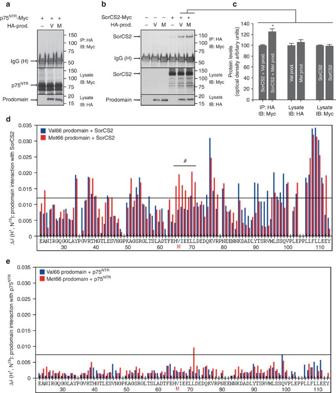Figure 6:The Val66 and Met66 prodomains binds differently to SorCS2 but do not bind to p75NTR. (a,b) HEK293T cells were transfected with the indicated constructs, the lysates were immunoprecipitated with anti-HA antibody, followed by detection with indicated antibodies. V=Val66 prodomain and M=Met66 prodomain constructs. (a) We were unable to detect interaction of either prodomains with p75NTRby co-immunoprecipitation. Representative blot of four independent experiments. (b) Both Val66 and Met66 prodomains co-immunoprecipitated with SorCS2; however, Met66 prodomain interacted ~23% more than the Val66 as quantified in (c). (c)n=9 independent experiments. Bars represent mean±s.e.m. Statistical comparisons were made by one-way analysis of variance test. *P<0.05. Interaction of Val66 and Met66 prodomains with SorCS2 (d) or p75NTR(e) was also assessed by NMR spectroscopy. Δδ= chemical shift deviation between Val66 and Met66 prodomains together with the receptors. Interaction of the prodomain with SorCS2 (d) was assessed at 4.5 μM for both proteins and data were collected at 600 MHz. The Met66 prodomain displayed greater chemical shift changes upon interaction to SorCS2 between residues 65 and 71 (shown under #) compared with the Val66 prodomain. Interaction of the prodomain with p75NTR(e) was assessed at 6.6 μM for both proteins and data were collected at 800 MHz. Interaction of the prodomain with p75NTRwas undetectable by NMR. Standard deviation (s.d.) was calculated for all the analysis and a threshold line equivalent to 2 s.d. was drawn to show the limit of what is considered interaction. Figure 6: The Val66 and Met66 prodomains binds differently to SorCS2 but do not bind to p75 NTR . ( a , b ) HEK293T cells were transfected with the indicated constructs, the lysates were immunoprecipitated with anti-HA antibody, followed by detection with indicated antibodies. V=Val66 prodomain and M=Met66 prodomain constructs. ( a ) We were unable to detect interaction of either prodomains with p75 NTR by co-immunoprecipitation. Representative blot of four independent experiments. ( b ) Both Val66 and Met66 prodomains co-immunoprecipitated with SorCS2; however, Met66 prodomain interacted ~23% more than the Val66 as quantified in ( c ). ( c ) n =9 independent experiments. Bars represent mean±s.e.m. Statistical comparisons were made by one-way analysis of variance test. * P <0.05. Interaction of Val66 and Met66 prodomains with SorCS2 ( d ) or p75 NTR ( e ) was also assessed by NMR spectroscopy. Δδ= chemical shift deviation between Val66 and Met66 prodomains together with the receptors. Interaction of the prodomain with SorCS2 ( d ) was assessed at 4.5 μM for both proteins and data were collected at 600 MHz. The Met66 prodomain displayed greater chemical shift changes upon interaction to SorCS2 between residues 65 and 71 (shown under #) compared with the Val66 prodomain. Interaction of the prodomain with p75 NTR ( e ) was assessed at 6.6 μM for both proteins and data were collected at 800 MHz. Interaction of the prodomain with p75 NTR was undetectable by NMR. Standard deviation (s.d.) was calculated for all the analysis and a threshold line equivalent to 2 s.d. was drawn to show the limit of what is considered interaction. Full size image To further confirm association of the Val66 or Met66 prodomains with SorCS2, we performed diffusion NMR measurements. Measurements of translational diffusion are highly sensitive to changes in hydrodynamic shape, which can be influenced by changes in intramolecular conformation and intermolecular associations. Association of the prodomains (10.2 kDa) with the ectodomain of SorCS2 (113 kDa) will influence the prodomain solution mobility and the apparent radius of hydration. The measured diffusion rates of Val66 and Met66 prodomains were 1.02 × 10 − 10 m 2 s − 1 and 1.04 × 10 − 10 m 2 s − 1 , respectively. Upon addition of SorCS2, Val66 display a slight decrease in diffusion D T Val66 =0.99 × 10 − 10 m 2 s − 1 , whereas the Met66 displayed significant reduction in diffusion rates to D T Met66 =0.74 × 10 − 10 m 2 s − 1 , corresponding to more than a doubling of the apparent hydrodynamic volume ( Supplementary Table S1 ). This indicates that the Met66 prodomain interacts with SorCS2 in a greater temporal extent as compared with the Val66 prodomain, and confirms that the Val66 and Met66 prodomains interact differentially with SorCS2. We could not detect significant structural changes in SorCS2 after either prodomain binding using intrinsic tryptophan fluorescence spectroscopy. Using tryptophan excitation at 285 nm, emission spectra with maxima at 329 nm was collected with SorCS2 alone as a control. The addition of Val66 or Met66 prodomain to SorCS2 showed emission maxima at 329 nm of 98.1 and 97.1% of the control, respectively. This is consistent with the lack of structural changes in Sortilin after neurotensin binding [26] . Significant chemical shift changes of either prodomain were not observed after the addition of p75 NTR by NMR ( Fig. 6e , Supplementary Fig. S9c,d ) confirming the lack of binding found by co-immunoprecipitation analysis. In contrast to the isolated prodomains, proBDNF was able to interact with SorCS2 and p75 NTR assessed by co-immunoprecipitation analysis ( Supplementary Fig. S7b ). SorCS2 is required for Met66-induced growth cone retraction As the prodomains interact with SorCS2, we evaluated whether SorCS2 is involved in Met66 prodomain-induced retraction of growth cones. To address this, we pre-incubated the hippocampal cultures with function-blocking antibodies directed against the SorCS2 ectodomain before the addition of the ligands. Addition of antibodies did not affect neuronal morphology, but blocked the ability of the Met66 prodomain to induce growth cone retraction ( Fig. 7a ). Control immunoglobulin Gs did not impair the effect ( Fig. 7a ). Moreover, anti-SorCS2 antibodies also blocked the ability of proBDNF to induce growth cone retraction ( Supplementary Fig. S7a ). To further confirm the involvement of SorCS2 in growth cone retraction triggered by the Met66 prodomain, we infected the hippocampal cultures with lentivirus expressing small hairpin RNA (shRNA) targeting SorCS2. SorCS2 shRNA expression resulted in a partial but significant decrease in SorCS2 protein levels as compared with the scrambled shRNA infection ( Fig. 7b ). The infection with scrambled shRNA resulted in higher growth cone retraction in basal conditions without ligand addition ( Fig. 7c ). However, the shRNA-induced SorCS2 decrease resulted in reduced growth cone retraction after Met66 prodomain administration, a result that is in agreement with the effects of function-blocking SorCS2 antibody experiments. 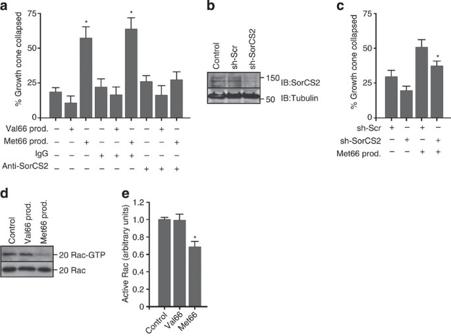Figure 7: Met66-SorCS2 interaction is required to induce growth cone retraction. (a) SorCS2 antibodies were able to block the Met66 prodomain-induced growth cone retraction. Neurons were pre-incubated with anti-SorCS2 (or control immunoglobulin Gs), treated with Val66 or Met66 prodomains (10 ng ml−1) for 20 min, and followed by growth cone retraction analysis. Quantification assessed in p75NTRpositive cells from three independent experiments. (b) Representative blot showing SorCS2 expression in cultured hippocampal neurons after knock-down using SorCS2 shRNA (sh-SorCS2) lentivirus infection, as compared with uninfected controls or scrambled shRNA (sh-Scr)-infected cells. (c) SorCS2 partial downregulation achieved with SorCS2 shRNA was able to partially prevent the Met66 prodomain-induced growth cone retraction. Quantification of four independent experiments. (d) Only Met66 prodomain administration, but not the Val66, induced a decrease in Rac activity in cultured hippocampal neurons. The hippocampal neurons were incubated with Val66 or Met66 prodomain for 20 min, and cell lysates were incubated with GST–PAK-CRIB beads to isolate activated Rac (Rac-GTP). (e) Quantification of (d). Activated Rac was measured by densitometry and normalized to total Rac in the input. Quantification assessed in four independent experiments. Bars represent mean±s.e.m. Statistical comparisons were made by one-way analysis of variance test. *P<0.05. Figure 7: Met66-SorCS2 interaction is required to induce growth cone retraction. ( a ) SorCS2 antibodies were able to block the Met66 prodomain-induced growth cone retraction. Neurons were pre-incubated with anti-SorCS2 (or control immunoglobulin Gs), treated with Val66 or Met66 prodomains (10 ng ml −1 ) for 20 min, and followed by growth cone retraction analysis. Quantification assessed in p75 NTR positive cells from three independent experiments. ( b ) Representative blot showing SorCS2 expression in cultured hippocampal neurons after knock-down using SorCS2 shRNA (sh-SorCS2) lentivirus infection, as compared with uninfected controls or scrambled shRNA (sh-Scr)-infected cells. ( c ) SorCS2 partial downregulation achieved with SorCS2 shRNA was able to partially prevent the Met66 prodomain-induced growth cone retraction. Quantification of four independent experiments. ( d ) Only Met66 prodomain administration, but not the Val66, induced a decrease in Rac activity in cultured hippocampal neurons. The hippocampal neurons were incubated with Val66 or Met66 prodomain for 20 min, and cell lysates were incubated with GST–PAK-CRIB beads to isolate activated Rac (Rac-GTP). ( e ) Quantification of ( d ). Activated Rac was measured by densitometry and normalized to total Rac in the input. Quantification assessed in four independent experiments. Bars represent mean±s.e.m. Statistical comparisons were made by one-way analysis of variance test. * P <0.05. Full size image Growth cones are rich in actin filament-containing structures such as lamellipodia and filopodia. The dynamic extension and retraction of these actin structures are regulated by Rho GTPases family members including Rac [27] . We previously showed that proNGF induces displacement of the guanine nucleotide exchange factor Trio from p75 NTR and SorCS2, thereby decreasing local activity of Rac to induce growth cone retraction [16] . To determine whether the Val66 prodomain, the Met66 prodomain or proBDNF lead to differential signalling downstream of SorCS2, we isolated and quantified activated Rac using the Cdc42/Rac interactive binding (CRIB) domain of the Rac effector p21-activated kinase (PAK-CRIB). Surprisingly, the Met66 prodomain or proBDNF exposure led to a significant decrease in Rac activity in the cultured hippocampal neurons, as compared with the absence of effect in Val66 prodomain-treated or in untreated neurons ( Fig. 7d,e ; Supplementary Fig. S7c ). The results strongly suggest that the helical preference in the Met66 prodomain is advantageous in interacting with SorCS2 and inducing active binding that is reflected in downregulation of Rac activity and growth cone retraction. In contrast, the Val66 prodomain with β-structure tendency remains inactive. We found that the variant Met66 prodomain acutely alters neuronal morphology, as it induces growth cone retraction. Mechanistically, we showed that the Val66Met substitution induces a shift in transient secondary structure from β-sheet to a helical conformation in the residues surrounding the substitution. This shift confers bioactivity to the Met66 prodomain through differential interaction with SorCS2, the sortilin-related Vps10p-domain sorting receptor 2. Moreover, we have demonstrated that the BDNF prodomain is detectable at high levels in vivo and that it is secreted in an activity-dependent manner from the cultured hippocampal neurons. In previous studies, the isolated BDNF prodomain was undetectable [10] . It is known that low-molecular-weight proteins can be detected more efficiently by cross-linking the peptides to the transfer membrane using glutaraldehyde [28] , [29] . Glutaraldehyde fixation of the proteins to the transfer membrane following SDS–PAGE and the use of a prodomain-specific monoclonal antibody previously characterized [10] , allow reliable detection of the prodomain in the murine central nervous system. However, we cannot rule out the possibility that the fixative promotes an antigen retrieval effect unmasking the prodomain epitopes. We corroborate that both the intracellular and the secreted prodomains are N -linked glycosylated as predicted by the amino-acid sequence. Furthermore, the developmental production of the prodomain parallels the expression of mBDNF [10] , [30] , [31] . The hippocampal expression of the prodomain in the Bdnf Met/Met mice is less than the observed in control Bdnf Val/Val mice, which is in agreement with a prior study that reported diminished hippocampal BDNF expression for the Bdnf Met/Met mice by enzyme-linked immunosorbent assay [32] . The Val66Met polymorphism leads to a decrease in the trafficking of BDNF to secretory vesicles and the subsequent impairment of activity-dependent release of BDNF [2] , [17] , [18] . The decreased levels of prodomain could in part be due to decreased transport and/or secretion from afferent inputs to the hippocampus such as the cortex or sub-cortical areas. Alternatively, it was reported previously that the Met66 BDNF transcripts show decreased dendritic trafficking [33] , and this may result in decreased local translation and secretion in the hippocampus. We cannot exclude the possibility that the Met66 proBDNF precursor exhibits decreased cleavage to its mature counterpart and prodomain, or that there is preferential degradation of the Met66 prodomain. Nonetheless, we were able to detect the Met66 prodomain in the Bdnf Met/Met mice hippocampus indicating that it may exert local bioactivity. Both mBDNF [34] and proBDNF [10] , [11] are secreted in an activity-dependent manner. Similarly, here we demonstrate that the release of the prodomain from neurons is also regulated by activity. Inhibition of extracellular cleavage of secreted proBDNF using α-2 anti-plasmin and an inhibitor of numerous matrix metalloproteinases did not significantly change the levels of the secreted prodomain in our culture conditions, suggesting that most of the cleavage of proBDNF to prodomain and mBDNF may occur in intracellular compartments. It has been reported that there is impaired regulated secretion of mBDNF from Bdnf Met/Met neuronal cultures [6] . In agreement with these studies, we found that there is a significant decrease in the activity-dependent release of the endogenous Met66 prodomain as compared with the Val66 prodomain. However, regardless of the secreted levels, both are detected in the media suggesting that they may act as ligands for paracrine or autocrine signalling. The Val66 and Met66 prodomains were determined to be intrinsically disordered with transient structural features using both NMR and CD spectroscopy. We detected specific conformational changes in the residues neighbouring the Val66Met substitution area, from β-structure propensity in the Val66 prodomain to helical conformation tendency in the Met66. It is known that small changes in local structure can substantially alter protein activity. This is particularly true in the case of intrinsically disordered proteins, which have prominent roles in signal transduction, antigen–antibody recognition, intracellular trafficking and as hormones, as well as in a number of neurodegenerative diseases such as Alzheimer’s, Huntington’s, Parkinson’s, prion and frontotemporal dementia diseases [35] , [36] . For instance, structural changes of similar magnitude to the ones observed for Val66Met substitution are observed in the A53T substitution in α-synuclein, which has been correlated to impact the kinetics of aggregation of this protein and toxicity in Parkinson’s disease [37] . The structural changes between Val66 and Met66 prodomain impact on their interaction with SorCS2 receptor, as the Met66 with more helical propensity, shows greater local chemical shifts perturbation during binding. We document that both Val66 and Met66 prodomains interact with SorCS2; however, they engage differentially as observed by NMR ( Fig. 6d ). Residues 65–71 of the Met66 prodomain interact with SorCS2, whereas the same residues in the Val66 prodomain do not engage the receptor, and this represents a novel region of interaction in the prodomain that is conferred by the Met66 substitution. This differential binding can explain the different bioactivity between the prodomains; however, other differences such as differential aggregation, bio-availability of the prodomains, differential trafficking or interaction of the prodomains with unknown factors may also have a role. This differential binding was confirmed by NMR diffusion measurements and co-immunoprecipitation experiments, and resulted in Rac inactivation only after Met66 addition to the cultured neurons. The development, maturation and plasticity of neuronal networks rely on the emergence, path finding and retraction of neuronal processes. Alterations in synaptic network organization influence the occurrence and progression of neuropsychiatric disorders [19] , [24] , [38] . ProNGF has been recently identified to activate p75 NTR and SorCS2 to promote fascin phosphorylation and its dissociation from actin filaments resulting in neurite retraction [16] . ProBDNF is also able to induce growth cone retraction as shown in Supplementary Fig. S7a confirming previously published studies [15] . Here we describe that the Met66 prodomain is sufficient to initiate growth cone retraction. As shown by NMR, the Met66 prodomain engages differently with SorCS2, but not with p75 NTR . However, Met66 prodomain is only active in p75 NTR -expressing cells suggesting that p75 NTR acts in a complex with SorCS2 or is downstream of SorCS2. ProBDNF interacts with both SorCS2 and p75 NTR and induces growth cone retraction. This may contribute to the bioactivity of proBDNF in this assay, whereas the Val66 prodomain that binds in a disadvantageous manner to SorCS2 is inactive. In early postnatal ages both proBDNF and processed products (mBDNF and prodomain) are present in the hippocampus. During adulthood, mBDNF and the prodomain are the most abundant forms, whereas proBDNF levels are decreased [10] . From this, we can infer that the actions of proBDNF may predominate in early postnatal time points, but the actions of the prodomain may prevail during adulthood. Most growth factors are synthesized as precursors, and prodomains are thought to function primarily to promote protein folding, intracellular sorting or to shield the mature domain from receptors to limit bioavailability [39] . Here we have demonstrated that the endogenous BDNF prodomain is detected in the hippocampus, and is secreted in an activity-dependent manner from neurons. Most importantly, the evolutionarily recent SNP that results in the Val66Met substitution in the prodomain promotes growth cone retraction in hippocampal neurons with involvement of p75 NTR and binding to SorCS2, in contrast to inactive Val66 prodomain. A function of the Val66 prodomain remains to be elucidated and future studies with mature neuronal networks are required to understand other prodomain actions. The endophenotypes related to neuropsychiatric disorders associated with the Val66Met polymorphism have been linked with decreased sorting and secretion of BDNF, thus impairing neuronal differentiation and plasticity via reduced tropomyosin-related kinase B receptor activation [32] , [33] . Here we show that the Met66 prodomain is a newly identified ligand that selectively activates SorCS2 to acutely alter neuronal morphology, and we propose that this effect is an additional mechanism that contributes to altered neural plasticity in humans with the SNP. Animals C57BL/6 male mice from different ages (as specified in the figures and captions) were maintained with a 12-h light–dark cycle and with free access to water and food. Val66Met knock-in mice ( Bdnf Met/Met ) and WT ( Bdnf Val/Val ) were used as reported previously [6] . Briefly, the BDNF coding region was replaced by a targeting vector with the BDNF sequence with or without a point mutation (G196A), which was introduced to result in the Val66Met substitution. These BDNF knock-in alleles are regulated by the endogenous BDNF promoters. Heterozygous Bdnf Val/Met mice were intercrossed to yield Bdnf Val/Val , Bdnf Val/Met and Bdnf Met/Met offspring at Mendelian rates. Heterozygous Bdnf +/− mice ( Bdnf tm1Jae ) were purchased from The Jackson Laboratory (Bar Harbour, ME, USA). Sprague–Dawley pregnant rats and C57BL/6 pregnant mice were purchased from Taconic Farms (Hudson, NY, USA) and Charles River (Wilmington, MA, USA), respectively. Animal care was in accordance with Weill Medical College of Cornell University IACUC. SDS–PAGE and western blot Dissected hippocampi or HEK293T (ATCC, Manassas, VA, USA) cells were lysed in 1% triton X-100 (Sigma, St Louis, MO, USA), 1% nonidet P-40 (Roche, Indianapolis, IN, USA), 10% glycerol, in buffer Tris-buffered saline pH 7.4 supplemented with protease inhibitor cocktail (Sigma). Protein concentration was determined by Bradford (Bio-Rad, Hercules, CA, USA). For deglycosylation, 100 μg of lysates or 100 μl of conditioned media were incubated with 1 μl of N -glycanase (ProZyme, San Leandro, CA, USA) for 1 h at 37 °C. The lysates or conditioned media were run in SDS–PAGE, the proteins were transferred to a 0.45-μm polyvinylidene fluoride (PVDF) membrane (Millipore, Billerica, MA, USA), and the membranes were fixed with 2.5% glutaraldehyde (Sigma) in PBS pH 7.4 unless otherwise written. After blocking with 5% bovine serum albumin (BSA) in Tris-buffered saline with 0.1% Tween 20, membranes were incubated with the prodomain antibody [10] (mAb287, 1:2000, 12–16 h at 4 °C, GeneCopoeia, Rockville, MD, USA), anti-β tubulin (Sigma, 1:15000, 1 h at 20–25 °C) or anti-SorCS2 (R&D Systems, Minneapolis, MN, USA, 1:1000, 12–16 h at 4 °C) followed by anti-mouse horseradish peroxidase (HRP) secondary antibody (1:5,000 for prodomain, or 1:15,000 for β-tubulin, 1 h at 20–25 °C, Calbiochem-Millipore) or anti-sheep HRP (1:5,000 for SorCS2, 1 h at 20–25 °C, Calbiochem-Millipore). Bands were analysed by enhanced chemiluminescence (Amersham-GE, Pittsburgh, PA, USA), and the densitometry was analysed using ImageJ (1.45, NIH, Bethesda, MD, USA, http://rsbweb.nih.gov/ij/ ). Quantization was normalized to β-tubulin for each individual sample. Full gel scans are provided in Supplementary Fig. S10 . Hippocampal cultures for prodomain secretion analysis Primary hippocampal neurons were isolated from E18 Sprague–Dawley rat embryos. Neurons were dissociated with 0.05% trypsin at 37 °C for 20 min followed by trituration with fire-polished glass pipettes. Cells plated on poly- D -lysine (Sigma)-coated dishes were grown in Neurobasal medium (Gibco, Grand Island, NY, USA) containing B27, 1 mM pyruvate (Gibco), 2 mM glutamine (Gibco), and 10 mM 5-fluorodeoxyuridine (Sigma). From day 3 in vitro to day 6, α-2-anti-plasmin (100 μM, Calbiochem-Millipore) and/or MMP Inhibitor II (10 μM, Calbiochem-Millipore; MMP1 IC 50 =24 nM, MMP3 IC 50 =18.4 nM, MMP7 IC 50 =30 nM, and MMP9 IC 50 =2.7 nM.) were added to the cultures. DIV6 media was collected and protease inhibitor cocktail (Sigma) was added. For depolarization experiments, 25 mM KCl was added to the cultures for 6 h. To study the secretion of the endogenous Val66 and Met66 prodomains, we cultured hippocampal–cortical neurons from E18 pups obtained from Bdnf Met/+ x Bdnf Met/+ litters. Each pup dissected area was plated in a different well and genotyped as described [6] . Subsequently, depolarization and harvesting of the culture media were performed as described for rat hippocampal cultures above. LDH release assay Conditioned media (50 μl) from DIV6 neurons in culture (with or without depolarization with KCl) was harvested and analysed for LDH levels using a colorimetric assay following the manufacturer’s protocol (CytoTox 96; Promega, Madison, WI, USA). Expression and purification of recombinant BDNF prodomains The plasmid pET28 (Novagen, Madison, WI, USA) containing the gene of human BDNF prodomain Val66 or Met66 (amino acids 23–113 preceded by an N-terminal His-tag and SUMO) [40] , was transformed in BL21(DE3)pLysS competent cells (Invitrogen, Grand Island, NY, USA). Proteins were produced using the Marley media swap method for isotopic labelling ( 15 N and 13 C/ 15 N) of recombinant proteins [41] . Prodomain samples were purified using a nickel resin column (Ni-NTA, Invitrogen). SUMO was cleaved by Ulp-1 (His6 tagged) proteolysis. Subsequently, the sample was negatively selected in a second nickel resin column where the now untagged BDNF prodomain was obtained in the flow though fraction. The resulting protein was precipitated using acetone, resuspended and dialyzed in 50 mM NaH 2 PO 4 100 mM NaCl pH 7.0. The sample purity was assessed by SDS–PAGE using Coomassie blue and silver staining methods ( Supplementary Fig. S3 ). The prodomains concentrations were calculated using random-coil UV absorbance in water ( ε (280) =4,470 M − 1 cm − 1 ) [42] , and confirmed using the Bradford method. NMR spectroscopy NMR samples were prepared in 93% H 2 O/7% D 2 O, 50 mM NaH 2 PO 4 100 mM NaCl pH 7.0 at concentrations varying from 2 μM to 450 μM. NMR spectra were acquired on a Bruker Avance 500 MHz, a Varian INOVA 600 MHz spectrometer both at Weill Cornell Medical College, and a Bruker Avance 800 MHz spectrometer at the New York Structural Biology Center. The 600 MHz and 800 MHz spectrometers were equipped with triple-resonance cryogenic probes. The 500 MHz spectrometer was equipped with a BBO room temperature probe and NMR chemical shift assignments were performed at 7 °C. NMR data were processed using the software nmrPipe [43] and analysed using Sparky [44] . Secondary structure predictions based on the observed chemical shifts were performed using the SSP [22] and TALOS+ 23 programs. Chemical shift deviation: Δ δ =[(Δ δ 1 H) 2 +(0.153*Δ δ 15 N) 2 ] 1/2 , where Δ δ 1 H and Δ δ 15 N are the 1 H and 15 N chemical shifts change, and 0.153 is a weighting factor for 15 N shifts. Interaction of the prodomain with recombinant human SorCS2 (R&D Systems) was assessed at 4.5 μM for both proteins and data were collected at 600 MHz. Interaction of the prodomain with human recombinant p75 NTR (R&D Systems) was assessed at 6.6 μM for both proteins and data were collected at 800 MHz. Data were processed and analysed using Topspin software (Bruker Instruments version 2.1). Sequential backbone resonance assignments were achieved using standard three dimensional HNCO, HNCA, HN(CO)CA, HNCACB and CBCA(CO)NH resonance heteronuclear experiments [45] . NMR diffusion measurements Gradient diffusion measurements were acquired using the BPP-LED pulse sequence [46] at 500 MHz in a Bruker Avance spectrometer, at 25 °C. Samples were all run in a volume constricted Shigemi tube, using a 20-mm sample height between plunger and tube bottom, to minimize convection artifacts. Data were collected at 298 K using 32 gradient experiments with linearly increasing z -gradient strengths from 2 to 95% of the maximum 55.7 G cm −1 , while maintaining a constant 6 ms gradient delay over the 100 ms diffusion period. The hydrodynamic radius was calibrated using 10 mM dioxane as an internal standard [47] . The data were processed and analysed using Bruker topspin software version 2.1. The hydrodynamic radius is calculated using the Stokes–Einstein equation D T = k B T (6 πηR h ) − 1 where D T is the translational diffusion coefficient, k B is Boltzmann constant, T is temperature in Kelvin, η is the solvent viscosity and R h is the hydrodynamic radius, by using dioxane as an internal reference the radius can be calculated R h =( D T dioxane / D T ) R h dioxane , assuming R h diovane =2.12 Å. Intrinsic tryptophan fluorescence spectroscopy Fluorescence data were collected on a spectrophotometer (Photon Technology International) at 20 °C with measurements from 305 nm to 500 nm in 1 nm increments. SorCS2, Val66 prodomain and Met66 prodomain were used at 0.17 μM in 50 mM Tris, 100 mM NaCl pH 7.0. CD spectroscopy CD spectra were acquired on an Aviv 62DS (Aviv Associates, Lakewood, NJ, USA) CD spectropolarimeter, using a 0.1 cm path length cuvette with 30 μM prodomains in 10 mM NaH 2 PO 4 50 mM NaCl pH 7.0. The wavelength dependence of molar ellipticity, [θ], was monitored at 23 °C as the average of four scans, using a 5-s integration time with 1.0-nm wavelength increments. Spectra were baseline-corrected against buffer alone. Growth cone retraction assay Primary hippocampal neurons were isolated from E15 C57BL/6 mouse embryos. Neurons were dissociated with 0.05% trypsin (Gibco) at 37 °C for 8 min followed by trituration with fire-polished glass pipettes. Cells plated on poly- D -lysine (Sigma)-coated dishes were grown in Neurobasal medium (Gibco) containing B27 (Gibco) and 0.5 mM glutamine (Gibco). Val66 proBDNF was collected from supernatants of HEK293FT cells (ATCC) transfected with a construct encoding human proBDNF (furin cleavage site mutated: RR128AA). proBDNF concentration was estimated by western blot (using BDNF antibody from Santa Cruz) comparing with known concentrations of recombinant BDNF (PeproTech, Rocky Hill, NJ, USA). For the assay, we added 10 or 50 ng ml −1 of the Val66 prodomain, Met66 prodomain or proBDNF to hippocampal neurons for 20 min before fixation. In order to block SorCS2, we pre-incubated cells with anti-SorCS2 (20 μg ml −1 , R&D Systems) or control sheep IgG for 20 min on ice before addition of the prodomains or proBDNF at 37 °C. DIV3 neurons were fixed with ice-cold methanol for 10 min. Coverslips were blocked with 10% normal donkey serum, 2% bovine serum albumin and 0.25% fish skin gelatin in Tris-buffered saline for 30 min; incubated with anti-Actin (1:10,000, Sigma, clone AC-74; anti-p75 NTR 1:1,000, R&D Systems; both for 30 min at 20–25 °C); followed by secondary antibodies (anti-goat Alexa 488, and anti-mouse Alexa 555, 1:1,000, Invitrogen) mixed with Hoechst (1:10,000) for 30 min at 20–25 °C; and mounted with Mowiol488 (Calbiochem-Millipore). Cells were imaged with an LSM 510 laser-scanning confocal microscope (with a 40 × Plan Neofluor, numerical aperture 1.3 DIC oil immersion objective, Carl Zeiss, Oberkochen, Germany). Images were processed with LSM 510 software (Carl Zeiss) and ImageJ. Co-immunoprecipitation experiments in HEK293T cells HEK293T cells (ATCC) were grown in DMEM supplemented with 10% fetal bovine serum (Gibco) and penicillin–streptomycin. Cells were transfected using Lipofectamine 2000 (Invitrogen) with Myc-tagged p75 NTR (a kind gift of Dr. Phil Barker), Myc-tagged SorCS2, HA/Flag-tagged Val66 prodomain, HA/Flag-tagged Met66 prodomain (both prodomains constructs produced by PCR using human pcDNA3.1 proBDNF as a template), and/or proBDNF constructs. Forty-eight hours after transfection, cells were lysed, and protein concentration was determined by Bradford (Bio-Rad). Lysates were pre-cleared with protein A-sepharose (Sigma), immunoprecipitated using an HA antibody (Sigma), followed by protein A-sepharose resin (Sigma). Following SDS–PAGE, the membranes were incubated with Myc antibody (1:15,000, 1 h at 20–25 °C, Bethyl) followed by anti-rabbit HRP secondary antibody (1:15,000, 1 h at 20–25 °C, Calbiochem-Millipore), or with HA.11 antibody (1:10,000, 1 h at 20–25 °C, Covance) followed by anti-mouse HRP secondary antibody (1:10,000, 1 h at 20–25 °C, Calbiochem-Millipore). Lentiviral vectors and transduction Lentiviral plasmids (pLKO.1) containing shRNA against mouse SorCS2 (targeting sequence: 5′-CGCTGAACTCTCATAGAATCA-3′) and a scramble control were obtained from Open Biosystems Thermo Scientific (Waltham, MA, USA). Lentivirus was packaged by co-transfection of shRNA constructs with packaging plasmids pMD2.G and pCMV-dR8.9 using TransIT-LT transfection reagent (Mirus, Madison, WI, USA) into HEK293FT cells. Media was changed 24 h later, and the media supernatant was collected 48 h after transfection. Supernatants were filtered through a 0.45-μm filter and pelleted by centrifugation with PEG-it (System Biosciences, Mountain View, CA, USA). Pellets were resuspended in Neurobasal medium (Gibco). Mouse primary hippocampal neurons were infected on DIV0 and medium was changed the following day. Rac activity assay Rac activity assays were performed as described previously [48] . Briefly, DIV2 hippocampal neurons were stimulated with Val66 prodomain, Met66 prodomains or proBDNF (10 ng ml −1 ) for 20 min, and cells were lysed in lysis buffer supplemented with 10 mM MgCl 2 . Cleared lysates were incubated with glutathione S-transferase (GST) or GST–PAK-CRIB beads (20 μg per reaction) for 30 min at 4 °C. Isolated active Rac was analysed by western blot using a Rac1 antibody (Millipore, clone 23A8), and normalized to the input. GST and GST–PAK-CRIB proteins were expressed in BL21(DE3)pLysS cells (Invitrogen) followed by incubation with glutathione sepharose. The purity of the recombinant proteins was analysed by Coomassie blue staining. How to cite this article: Anastasia, A. et al. Val66Met polymorphism of BDNF alters prodomain structure to induce neuronal growth cone retraction. Nat. Commun. 4:2490 doi: 10.1038/ncomms3490 (2013).